Polymer collapse in miscible good solvents is a generic phenomenon driven by preferential adsorption Water and alcohol, such as methanol or ethanol, are miscible and, individually, good solvents for poly(N-isopropylacrylamide) (PNIPAm), but this polymer precipitates in water–alcohol mixtures. The intriguing behaviour of solvent mixtures that cannot dissolve a given polymer or a given protein, while the same macromolecule dissolves well in each of the cosolvents, is called cononsolvency. It is a widespread phenomenon, relevant for many formulation steps in the physicochemical and pharmaceutical industry, that is usually explained by invoking specific chemical details of the mixtures: as such, it has so far eluded any generic explanation. Here, by using a combination of simulations and theory, we present a simple and universal treatment that requires only the preferential interaction of one of the cosolvents with the polymer. The results show striking quantitative agreement with experiments and chemically specific simulations, opening a new perspective towards an operational understanding of macromolecular solubility. Stimuli-responsive polymers, often referred to as smart polymers, are macromolecular systems whose structure, function and stability are intimately linked to external parameters, such as temperature, external fields, ionic strengths or cosolvent concentrations [1] , [2] . This is the origin of the responsiveness of hydrogels exposed to external stimuli or concentration gradients [3] , [4] , [5] , [6] and denaturation of proteins [7] , [8] , [9] . One of the solvents is usually water, however, the responsiveness is not necessarily restricted to water-soluble polymers. While understanding the physical behaviour of smart polymers is theoretically challenging, they experience a wide variety of applications that range from biology to physics. For example, smart polymers can be used for bio-interfaces, sensors, regulating cell culture, drug delivery, artificial muscle tissue, surface adhesion and wetting, to name a few [1] , [10] , [11] . Thus, a more thorough and generally applicable understanding of their properties is highly desirable. Most common stimuli-responsive polymers display a transition from an extended coil structure at low temperature to a compact globule when temperature is increased, thus presenting a lower critical solution temperature (LCST). There are many examples of polymers that have a LCST, such as poly(N-isopropylacrylamide) (PNIPAm), poly(N,N-diethylacrylamide), poly(N-vinlycaprolactam), and/or poly(acryloyl- L -proline methyl ester) (PAPOMe), where PNIPAm is one of the most commonly known stimuli-responsive polymer. There has been long standing interest in studying PNIPAm in water and/or in mixed solvents by means of experiment [3] , [4] , [6] , [12] , theory [3] , [13] , [14] and computer simulation [15] , [16] , [17] . In pure water, PNIPAm has a LCST of 305 K [13] , [15] . Moreover, if methanol is added to the water as cosolvent, PNIPAm shows an interesting re-entrant coil–globule–coil transition with increasing methanol mole fraction x m [4] , [6] , [12] at ambient temperature. So does PAPOMe in aqueous methanol [18] . Furthermore, mixed solvents also play a role in completely different areas of soft-matter research and technology, such as organic electronics [19] . It has been observed that the solution viscosity of polymeric semiconductors can display a nonmonotonic dependency on cosolvent concentration, implying conformational changes of the polymer [19] and indicating that such phenomena are by no means restricted to the ‘so called’ stimuli-responsive polymers. Theoretical investigations typically concentrate on either a Flory–Huggins type analysis [3] , [20] or cooperative hydrogen-bonding effects [14] , while simulations usually deal with all-atom descriptions [15] , [16] . More recently, two of us have proposed a semi-grand canonical multi-scale approach to study PNIPAm in aqueous methanol and have shown that the coil–globule–coil transition can be linked to the delicate balance of intermolecular interactions between PNIPAm–methanol and PNIPAm–water [17] . The method considered chemical details only within the correlation length originating from the solute structure, which was coupled to a semi-grand canonical particle reservoir. The aim of this work is to propose a general concept for polymers in mixed solvents, which can account for the phenomenon of coil–globule–coil scenario in mixed (good) cosolvents. We show that due to the discrete nature of solute–(co)solvent coordination, mean-field-type arguments may not be sufficient to describe the conformational behaviour of stimuli-responsive polymers. Instead, a discrete-particle-based explanation is needed, which will be provided in this work. By this, we demonstrate that the origin of this swelling–collapse–swelling transition is generic and that many polymers can be expected to display similar conformational transitions, as long as there is a preferential coordination between the macromolecule and one of the cosolvents. Conformation of polymer We first demonstrate that our simple model is capable of reproducing the essentials of the experimentally observed re-entrant coil–globule–coil scenario of PNIPAm and PAPOMe in aqueous methanol [4] , [6] , [18] . In Fig. 1a , we summarize the radius of gyration R g as a function of cosolvent molar concentration x c , where we compare the data from the generic bead-spring model with the experimentally observed degrees of swelling q [6] , [18] and our previous multi-scale simulation results [17] . It can be appreciated that the generic model reproduces the characteristic swelling–collapse–swelling transition of polymers in mixed solvents. Even when both solvents are individually good solvents for the polymer, their combination causes the chains to collapse in the apparent poor solvent at a concentration range 0.1< x c <0.5. The simple model is even in particularly good agreement with the experimental data of PNIPAm. 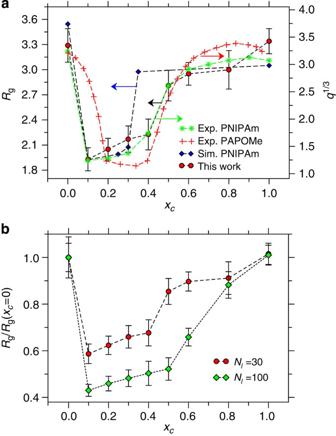Figure 1: Conformation of a polymer in mixed cosolvents and system size effect. Radius of gyrationRgas a function of cosolvent molar concentrationxc. The sizes of solventsand cosolventccomponents are chosen as 0.5σand the interaction well depth between polymerpandcis taken asεpc=1.0ε. (a) shows results for chain lengthNl=30. For comparison, we include data from the semi-grand canonical multi-scale simulations with all-atom details17. We also include experimental data obtained from the degree of volume swelling ratioqfor PNIPAm6and PAPOMe18. For representative purposes, the data from the multi-scale simulations and PAPOMe are shifted. The arrows indicate the correspondingyaxis. (b) showsRg/Rg(xc=0) as a function ofxcfor two different chain lengthsNl. In both parts, the error bars are the s.d. calculated from six independent simulations. The lines are drawn to guide the eye. Figure 1: Conformation of a polymer in mixed cosolvents and system size effect. Radius of gyration R g as a function of cosolvent molar concentration x c . The sizes of solvent s and cosolvent c components are chosen as 0.5 σ and the interaction well depth between polymer p and c is taken as ε pc =1.0 ε . ( a ) shows results for chain length N l =30. For comparison, we include data from the semi-grand canonical multi-scale simulations with all-atom details [17] . We also include experimental data obtained from the degree of volume swelling ratio q for PNIPAm [6] and PAPOMe [18] . For representative purposes, the data from the multi-scale simulations and PAPOMe are shifted. The arrows indicate the corresponding y axis. ( b ) shows R g / R g ( x c =0) as a function of x c for two different chain lengths N l . In both parts, the error bars are the s.d. calculated from six independent simulations. The lines are drawn to guide the eye. Full size image The initial collapse transition on adding cosolvent is sharp and suggests a first-order-like scenario. Indeed, there are no indications of an extended blob structure known from a conventional Θ-collapse. Taking the degree of shrinking from Fig. 1b , we get [ R g / R g ( x c =0, N =30)]/[ R g / R g ( x c =0, N =100)] ≅ 0.43 as expected for a good solvent coil to dense globule transition. More details of R g as a function of N l for coil and globule conformations are presented in the Supplementary Note 1 and Supplementary Fig. 1 . In contrast, on further addition of (better) cosolvent between 0.5< x c <0.8, the polymer starts to expand again towards the fully expanded coil, however, in a much more gradual, certainly not first-order-like manner. The transition appears significantly shifted towards higher cosolvent concentration for N =100 and, contrary to normal critical phenomena, even somewhat smoother. To understand this counter-intuitive behaviour, we will come back to this scenario at a later stage. Chemical potential of polymer So far we have demonstrated that the generic model correctly reproduces the coil–globule–coil scenario. It, however, also reproduces a striking similarity of intermolecular affinity known from chemically specific system of PNIPAm in aqueous methanol [17] (for more details see Supplementary Fig. 2 in Supplementary Note 2 ). Therefore, thermodynamic properties, such as the chemical potential of polymer μ p that is intimately linked to relative (co)solvent interactions, should also display similarity with the all-atom data. A classic theory that connects intermolecular affinities in a solution to its thermodynamic properties is the fluctuation theory of Kirkwood and Buff [21] . If a polymer, p, at dilute concentration is solvated in a mixture of solvent s and cosolvent c , μ p can be calculated using [22] , where , and ρ c is the cosolvent number density. G ij is the Kirkwood–Buff integral that is related to the pair distribution function g ij ( r ) via . The integration of equation 1 gives a direct estimate of the shift in with increasing x c . In Fig. 2 , we show a master plot of as a function of x c . It can be appreciated that the data from a simple generic model are in reasonably good agreement with the data obtained from the simulations incorporating chemical details. The agreement is particularly striking within the range 0.1< x c <0.5 when the polymer collapses into a globule. Furthermore, a more detailed analysis of equation 1 suggests that for an ideal model case, when G cs = G cc , factor 1− ρ c ( G cs − G cc )=1. In all-atom descriptions of aqueous methanol, 1.0≤1− ρ c ( G cs − G cc )≤1.1 (ref. 17 ). This makes the denominator in equation 1 invariant, within the stochastic error bar, between 0.1< x c <0.5. Therefore, the shift in is dominated by G ps − G pc and the good agreement in Fig. 2 further suggests that the bead-spring model could capture the correct relative intermolecular affinity, which is an important factor in the occurrence of the re-entrant coil–globule–coil transition in mixed solvents. It is yet important to emphasize that the striking quantitative similarity between the generic simulation and the all-atom data is only made possible because of the comparable energy scale in both cases, which is of the order of 2 κ B T . 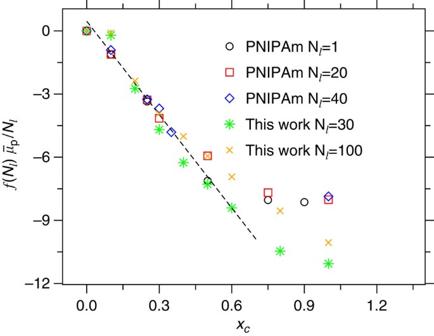Figure 2: Thermodynamics of polymer collapse. Chemical potential shiftper monomer as a function of cosolvent mole fractionxc.obtained from the generic model is compared with the data from the atomistic configuration of PNIPAm, which is taken from ref.17. The master curve is obtained by normalizing thewith a chain lengthNl-dependent functionf(Nl)=2Nl/(Nl+1) (seeSupplementary Note 3). Figure 2: Thermodynamics of polymer collapse. Chemical potential shift per monomer as a function of cosolvent mole fraction x c . obtained from the generic model is compared with the data from the atomistic configuration of PNIPAm, which is taken from ref. 17 . The master curve is obtained by normalizing the with a chain length N l -dependent function f ( N l )=2 N l /( N l +1) (see Supplementary Note 3 ). Full size image Another striking aspect of the variation in is that even when the polymer collapses into a compact globular structure, within the range 0.1< x c <0.5, systematically decreases with increasing x c . Ideally, within a mean-field-type description, such as the Flory–Huggins theory [3] , one expects an increase in when the polymer first collapses around x c ≈0.1, then starts to decrease again for x c >0.5, see Supplementary Fig. 3 . Here, however, we see a distinctly different behaviour, making the mean-field-type description highly unsuitable for understanding these complex discrete-particle-based phenomena. Therefore, a theoretical framework is needed where the particle-based preferential binding scenario can be incorporated. This is lacking in the literature and will be proposed below. We now develop a generic microscopic picture of the polymer conformation in mixed solvents. The compact globular structure is driven by the preferential attraction of cosolvent to the polymer. At low cosolvent concentration x c →0, c molecules can bind to two distinctly far monomers inducing bridges that initiate the collapsing process. At high concentrations, when a large number of c molecules is added ( x c →1) they decorate the polymer and allow for the extended coil structure. In Fig. 3 , we show simulation snapshots during polymer collapse for N l =100. 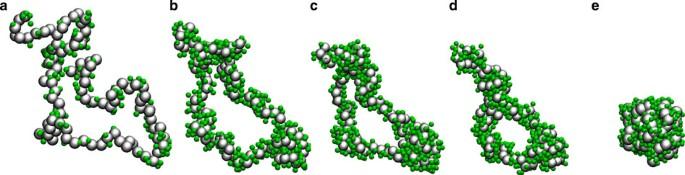Figure 3: Polymer collapse dynamics. Simulation snapshots showing dynamics of polymer collapse for chain lengthNl=100 and at at a cosolvent mole fractionxc=0.1. Cosolvent particles are drawn within unity distance from the polymer. Snapshots are rendered at different timesτof production run: (a)t=100τ, (b)t=100τ, (c)t=750τ, (d)t=1,250τand (e) final globular conformation, allowing for a ‘release’ of cosolvent particles. Similar behavior is observed for every case of globule conformation. However, for the clarity of representation, we choosexc=0.1. Figure 3: Polymer collapse dynamics. Simulation snapshots showing dynamics of polymer collapse for chain length N l =100 and at at a cosolvent mole fraction x c =0.1. Cosolvent particles are drawn within unity distance from the polymer. Snapshots are rendered at different times τ of production run: ( a ) t =100 τ , ( b ) t =100 τ , ( c ) t =750 τ , ( d ) t =1,250 τ and ( e ) final globular conformation, allowing for a ‘release’ of cosolvent particles. Similar behavior is observed for every case of globule conformation. However, for the clarity of representation, we choose x c =0.1. Full size image It is apparent that the polymer collapse is initiated by several patches along the backbone. A significant Ω-type loop is visible at t =300τ ( Fig. 3b ) before finally collapsing into a compact globule ( Fig. 3e ). From Fig. 3 , it is also evident that one can distinguish two types of cosolvent molecules among those that decorate the polymer. A fraction φ B forms bridges between two (distinctly far) monomers and a fraction φ binds to one monomer only. In the collapsed state, one expects to see an increased value of φ B . On the other hand when the polymer re-opens, bridging should vanish φ B →0. In Fig. 4a , we show φ B as a function of x c for N l =100. As expected, the data (red stars) show a distinct hump between 0.1< x c <0.5 consistent with the collapsed conformation observed in Fig. 1 . 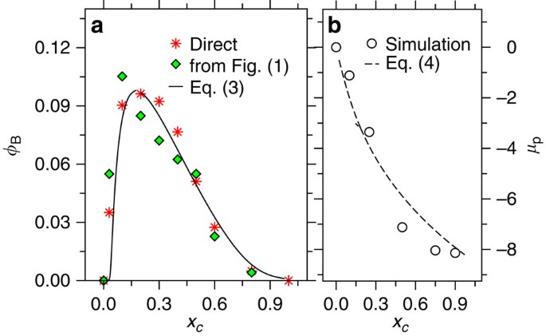Figure 4: Comparison of theory with computer simulations. (a) shows bridging fraction of cosolventsφBas a function of methanol mole fractionxcforNl=100. The data corresponding to red stars is the direct calculation ofφBfrom the simulation trajectory. For comparison, we have also shown the effective negative excluded volume, which can be calculated using the expression [{Rg/Rg(xc=0)}−3−1] (see green diamonds). HereRg/Rg(xc=0) is taken fromFig. 1b. The prediction of analytical theory from equation 3 is plotted as solid line.bshows chemical potential of a single monomerμpas a function ofxc. We also include the analytical expression in equation 4. Figure 4a also shows that the strength of the effective negative excluded volume (green diamonds), extracted from the inverse variation of the gyration radius −≈[{ R g / R g ( x c =0)} −3 −1], is proportional to φ B . Figure 4: Comparison of theory with computer simulations. ( a ) shows bridging fraction of cosolvents φ B as a function of methanol mole fraction x c for N l =100. The data corresponding to red stars is the direct calculation of φ B from the simulation trajectory. For comparison, we have also shown the effective negative excluded volume, which can be calculated using the expression [{ R g / R g ( x c =0)} −3 −1] (see green diamonds). Here R g / R g ( x c =0) is taken from Fig. 1b . The prediction of analytical theory from equation 3 is plotted as solid line. b shows chemical potential of a single monomer μ p as a function of x c . We also include the analytical expression in equation 4. Full size image Using the information in Fig. 4a , we can now explain why we observe a smoother re-swelling for N l =100 ( Fig. 1b ). It is evident that at x c =0.5 and 0.6, there are still a significant fraction of bridging cosolvents present, thus leading to a somewhat semi-collapsed and/or semi-extended structure. However, for N l =30, we find vanishing φ B between 0.5< x c <0.8 (data not shown) consistent with the fully extended structure. This observation is not surprising, given that the longer polymers have larger flexibility to form small segmental loops. Within a simple scaling argument, the loop formation can be characterized by the partition function of vanishing end-to-end distance R e →0, which reads . Here 1/ Q is the critical fugacity and the universal exponent α ≈0.2 [23] . Furthermore, the partition function at finite R e is given by with γ =1.15 [23] , [24] . From these two cases, one can estimate the free-energy barrier to form a loop of length N l as Δ( N l )= mκ B T ln( N l ), with m = γ − α +1≈1.95 being the critical exponent [23] . For the segmental loop formation of length n , one can use the same expression as Δ(n)= mκ B T ln( n ). Therefore, this argument leads to an energy penalty for the loop formation, shown above, that is of the order of κ B T . Numerical simulation results thus show that the preferential adsorption of cosolvents onto the chain backbone controls both collapse and re-swelling of the polymer. This is the opposite of mean-field polymer theories, where polymer phase behaviour is dictated by the average field of cosolvent, irrespective of its spatial distribution within the solvation volume spread by the polymer chain. A simple theoretical description of cononsolvency can thus be formulated by considering the fractions φ B and φ of cosolvent adsorbed onto the polymer backbone, while the remaining fraction of adsorption sites 1− φ B − φ is occupied by the solvent molecules. The adsorption free energy per unit adsorption site reads, where the first three terms in the right-hand side are entropic contributions, the factor 2 in the term for the mixing entropy accounts for the fact that a bridge occupies two sites on the polymer backbone, and the next two terms correspond to the adsorption energies B and that measure the excess affinities of individual bridging and non-bridging cosolvent molecules to the chain backbone. μ = κ B T ln( x c ) is the chemical potential of the cosolvent in the bulk solvent mixture. Crucially, one recognizes that the bridging affinity B is reduced with respect to 2 by the cost of loop formation, , where and n =1/ φ B . Minimization of equation 2 with respect to φ B and φ (that is, solving ∂Ψ/∂ φ =∂Ψ/∂ φ B =0) results in an analytical relation between φ B and x c , which reads where and . The solution of equation 3 is shown as a solid line in Fig. 4a with m =1.95 as expected [23] and consistent with the bridging scenario. Not only does the theory show a striking similarity with the simulation data, but it also quantitatively predicts the variation of μ p as a function of x c , as shown in Fig. 4b . In summary, we have performed molecular dynamics simulations of a generic bead-spring model to study the coil–globule–coil transition of macromolecules in mixed solvents. Though the simulation protocol is completely independent of chemical details, the simulations show striking quantitative agreement with the experimental data of PNIPAm and PAPOMe in aqueous methanol. Additionally, the simplified model also shows striking agreement with the competitive coordination of polymer known from the all-atom descriptions. This suggests that the origin of these complex, cosolvent-driven, conformational transitions is generic in nature and does not depend on the specific chemical details. Therefore, a broad range of polymeric systems are expected to demonstrate similar re-entrant behaviour, so long as there is a preferential cosolvent binding. This, however, does not mean that the solvent quality becomes poor, contrary to what is known from the present understanding. Instead, a polymer even collapses in a mixed ‘good’ solvent because of the preferential binding. Such discrete-particle-based phenomena cannot be explained with a mean-field-type picture. Therefore, we here propose a theoretical description based on the selective adsorption of the cosolvent with the polymer backbone that can describe the numerical results. We find that the coil–globule–coil scenario can be understood by the segmental loop formation, facilitated by the bridging cosolvents connecting two monomers that are far from one another along the backbone. The theory also helps to understand the counter-intuitive system size effect, namely the longer the chain the smoother the re-swelling transition at larger cosolvent concentrations. Usually, our simulations deal with one thermodynamic state point of temperature in a mixture of cosolvents and not with the temperature-induced polymer collapse. Furthermore, we would like to point out that although our results are compared and presented in the context of thermoresponsive polymers that have a LCST, such as PNIPAm and PAPOMe [13] , [15] , [18] , our findings are not restricted to these polymers, another classical example includes polymeric semiconductors [19] . Therefore, our results present a simple, yet effective, insight into the solubility behaviour of polymer and proteins, paving the ways for the development of accurate methods to control co(non)solvency in an applied environment. Molecular dynamics simulations We have used the well-known bead-spring polymer model [25] . In this model, individual monomers of a polymer interact with each other via a repulsive 6–12 Lennard-Jones (LJ) potential, where ε p =1.0 ε and σ p =1.0 σ . All units are expressed in terms of the LJ energy ε , the LJ radius σ and the mass m of individual particles. This leads to a time unit of . Additionally, adjacent monomers in a polymer are connected via a finitely extensible nonlinear elastic potential, where R 0 =1.5 σ and k =30 ε / σ 2 . The parameters of the potential are such that a reasonably large time step can be chosen, while bond crossing remains unlikely to occur. A bead-spring polymer p is solvated in mixed solutions composed of two components also modelled as LJ beads, solvent s and cosolvent c , respectively. Note that for the study of macromolecules in aqueous methanol, the water molecules are referred as solvent and the methanols as cosolvent. Since the solvent molecules are much smaller than the monomers of PNIPAm and/or PAPOMe in aqueous methanol, we choose the size of solvents to be σ s/c =0.5 σ and the size of the monomers is σ p =1.0 σ . Based on the Kirkwood–Buff analysis of PNIPAm in aqueous methanol [17] , the system is set in such a manner that the two solvents are perfectly miscible, that is, they do not experience each other as different, while c is a somewhat better solvent than s . This is done by choosing the interactions between p and s to be a repulsive LJ potential, with ε ps =1.0 ε and σ ps =0.5 σ . The p − c interaction uses a full LJ potential, Unless stated otherwise, the interaction well depth between p and c is chosen as ε pc =1.0 ε with σ pc =0.75 σ . Solvent particles always repel each other with the same repulsive LJ, with ε ij =1.0ε and σ ij =0.5 σ . This is a good approximation given that the p − c interaction is dominant over s − s , s − c and c − c interactions. For more details, see the comparison of all-atom and experimental data presented in Supplementary Fig. 4 and the corresponding discussion in Supplementary Note 4 . The cosolvent mole fraction x c is varied from 0 (pure s component) to 1 (pure c component). We consider two different polymer chain lengths N l =30 and 100, solvated in 2.5 × 10 4 solvent molecules for N l =30 and 10 × 10 4 solvent molecules for N l =100, respectively. The equations of motion are integrated using a velocity Verlet algorithm with a time step δt =0.005 τ and a damping coefficient Γ=1.0τ −1 for the Langevin thermostat, with the temperature set to T =0.5 ε / κ B , where κ B is the Boltzmann constant. The initial configurations are equilibrated for typically several 10 5 τ , depending on the chain length, which is at least an oder of magnitude larger than the relaxation time in the system. After this initial equilibration averages are taken over another 10 4 τ to obtain observables, especially gyration radii R g , chemical potentials μ p of the polymer and the bridging fractions of cosolvents φ B . Simulations are performed using ESPResSo++ molecular dynamics package [26] and the snapshots in this manuscript are rendered using VMD [27] . How to cite this article: Mukherji, D. et al . Polymer collapse in miscible good solvents is a generic phenomenon driven by preferential adsorption. Nat. Commun. 5:4882 doi: 10.1038/ncomms5882 (2014).